Ultrafast collinear scattering and carrier multiplication in graphene Graphene is emerging as a viable alternative to conventional optoelectronic, plasmonic and nanophotonic materials. The interaction of light with charge carriers creates an out-of-equilibrium distribution, which relaxes on an ultrafast timescale to a hot Fermi-Dirac distribution, that subsequently cools emitting phonons. Although the slower relaxation mechanisms have been extensively investigated, the initial stages still pose a challenge. Experimentally, they defy the resolution of most pump-probe setups, due to the extremely fast sub-100 fs carrier dynamics. Theoretically, massless Dirac fermions represent a novel many-body problem, fundamentally different from Schrödinger fermions. Here we combine pump-probe spectroscopy with a microscopic theory to investigate electron–electron interactions during the early stages of relaxation. We identify the mechanisms controlling the ultrafast dynamics, in particular the role of collinear scattering. This gives rise to Auger processes, including charge multiplication, which is key in photovoltage generation and photodetectors. Photonics encompasses the generation, manipulation, transmission, detection and conversion of photons. Applications of photonics are nowadays ubiquitous, affecting all areas of everyday life. Photonic devices, enabled by a continuous stream of novel materials and technologies, have evolved with a steady increase in functionalities and reduction of device dimensions and fabrication costs. Graphene has decisive advantages [1] , such as wavelength-independent absorption, tunability via electrostatic doping, large charge-carrier concentrations, low dissipation rates, high mobility and the ability to confine electromagnetic energy to unprecedented small volumes [1] , [2] . These unique optoelectronic properties make it an ideal platform for a variety of photonic applications [1] , including fast photodetectors [3] , [4] , transparent electrodes in displays and photovoltaic modules [1] , optical modulators [5] , plasmonic devices [2] , [6] , microcavities [7] , ultrafast lasers [8] , to cite a few. Understanding the interaction of light with graphene is pivotal to all these applications. In the first instance, absorbed photons create optically excited (‘hot’) carriers. Their non-equilibrium dynamics can be very effectively studied by ultrafast pump-probe spectroscopy. In this technique, an ultrashort laser pulse creates a strongly out-of-equilibrium (non-thermal) distribution of electrons in conduction band and holes in valence band. The optically excited carriers then relax, eventually reaching thermal equilibrium with the lattice. The relaxation dynamics, due to various processes, including electron–electron (e–e) and electron–phonon (e–ph) scattering, as well as radiative electron–hole (e–h) recombination, is then accessed by a time-delayed probe pulse (see Fig. 1 ). The time-evolving hot-electron distribution inhibits, due to Pauli blocking, the absorption of the probe pulse at lower photon energies with respect to the pump, thus yielding an increase in transmission (‘photobleaching’ (PB)). Thus, monitoring this transient absorption enables the direct measurement of the distribution function in real time. Here we are interested in the early stages of the dynamics, during which two main processes occur: (i) the initial peak produced by the pump laser broadens, due to e–e collisions, converging towards a hot Fermi-Dirac (FD) shape in an ultrashort timescale [9] , [10] , [11] . (ii) Then, optical phonon emission [12] becomes predominant and drives a cooling in which the FD distribution shifts towards the Dirac point. 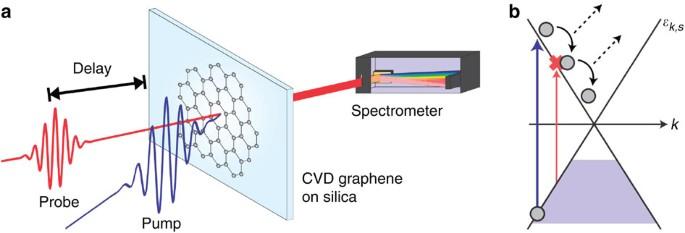Figure 1: Pump-probe set-up. (a) A pump and a probe pulse, with different colours, impinge on a sample with a variable delay. The spectrum of the probe pulse through the sample is measured by a spectrometer. (b) MDF bands in graphene, εk,s=sv|k| withs=±1 andm s−1. Pump (blue arrow) and probe pulses (red arrow) are applied at different photon energies in a hole-doped sample. The electron distribution relaxes towards the Dirac point by losing energy. Electrons (grey circles) transfer energy to other degrees-of-freedom (dashed arrows), such as phonons and other electrons in the Fermi sea. When half of the probe-pulse energy matches the maximum of the electron distribution, absorption is strongly suppressed by Pauli blocking (red cross) and the transition is ‘bleached’. Figure 1: Pump-probe set-up. ( a ) A pump and a probe pulse, with different colours, impinge on a sample with a variable delay. The spectrum of the probe pulse through the sample is measured by a spectrometer. ( b ) MDF bands in graphene, ε k , s = sv | k | with s =±1 and m s −1 . Pump (blue arrow) and probe pulses (red arrow) are applied at different photon energies in a hole-doped sample. The electron distribution relaxes towards the Dirac point by losing energy. Electrons (grey circles) transfer energy to other degrees-of-freedom (dashed arrows), such as phonons and other electrons in the Fermi sea. When half of the probe-pulse energy matches the maximum of the electron distribution, absorption is strongly suppressed by Pauli blocking (red cross) and the transition is ‘bleached’. Full size image In order to experimentally access the very first stages of relaxation and to disentangle the role of e–e scattering from other mechanisms, it is necessary to probe at an energy lower than that of the pump and , at the same time, achieve the highest possible temporal resolution. Pump-probe spectroscopy has been extensively employed to investigate relaxation processes in carbon-based materials: a variety of different samples have been studied, including thin graphite [13] , few- [14] , [15] , [16] and multi-layer [17] graphene, but very few did experiments on single-layer graphene (SLG) [18] , [19] , [20] , [21] . Furthermore, the temporal resolution reported in earlier literature, either in degenerate (i.e., pump and probe with same photon energy) or two-colour pump-probe, was in most cases ≥100 fs [14] , [15] , [16] , [17] , [18] , [21] . This prevented the direct observation of the intrinsically fast e–e scattering processes. The electron distribution in graphene was also mapped by time-resolved photoemission spectroscopy [22] ; however, its evolution on the critical sub-100-fs timescale was not resolved. Thus, earlier studies mostly targeted the phonon-mediated cooling of a thermalized (but still hot) electron distribution, established within the pump pulse duration. To date, only Breusing et al . [20] probed SLG with a resolution~10 fs. However, this was a degenerate experiment, probing the relaxation dynamics on a limited spectral window. The thrust of this work is to investigate the role of e–e interactions on the initial stages of the non-equilibrium dynamics. Even at equilibrium, e–e interactions are responsible for a wealth of exotic phenomena in graphene [23] . They reshape the Dirac bands [24] , [25] and substantially enhance the quasiparticle velocity [25] . Angle-resolved photoemission spectroscopy showed electron–plasmon interactions in doped samples [24] , and a marginal Fermi-liquid behaviour in undoped ones [26] . Many-body effects were also revealed in optical spectra both in the infrared (IR) [27] and in the ultraviolet [28] , where strong excitonic effects were measured [28] . In the non-equilibrium regime, an extremely fast e–e relaxation on a timescale of tens fs was theoretically suggested in refs 29 , 30 , 31 , 32 . However, these pioneering approaches relied solely on numerical methods and, as discussed below, did not take full advantage of the symmetries of the scattering problem. This resulted in an uncontrolled treatment of crucially important ‘collinear’ scattering events (i.e., with the scattering particles’ incoming and outgoing momenta on the same line), thus characterized by a high degree of symmetry. A deeper theoretical understanding of collinear scattering events and, most importantly, their phase space, requires more work. Here we combine extreme temporal resolution broadband pump-probe spectroscopy with a microscopic semi-analytical theory based on the semiclassical Boltzmann equation (SBE) to investigate e–e collisions in graphene during the very early stages of relaxation. We identify the fundamental processes controlling the ultrafast dynamics, in particular the significant role of Auger processes, including charge multiplication. Samples and pump-probe experiments SLG is grown by chemical vapour deposition (CVD) and transferred onto 100 μm quartz substrates (see Methods ). These are selected because they induce negligible artifacts in the pump-probe experiments, as further verified here by measuring the uncoated substrates (see Methods ). We perform two-colour pump-probe spectroscopy using few-optical-cycle pulses (see Methods ). We impulsively excite inter-band transitions with a 7 fs visible pulse at 2.25 eV (2–2.5 eV bandwidth) and probe with a 13 fs IR pulse (1.2–1.45 eV bandwidth), as well as a red-shifted 9 fs IR pulse (0.7–1.2 eV bandwidth). The density of photoexcited electrons is~10 13 cm −2 (see Methods ), while the equilibrium carrier density before photoexcitation corresponds to ~200 meV hole doping (see Methods ). The availability of such short IR probe pulses allows us to follow the electron population as it evolves towards a FD distribution. Our instrumental response function (full width at half maximum of the pump-probe cross-correlation) is <15 fs [33] , with a crucially important order of magnitude improvement compared with previous two-colour studies [16] , [17] . This allows us to directly probe the e–e dynamics. 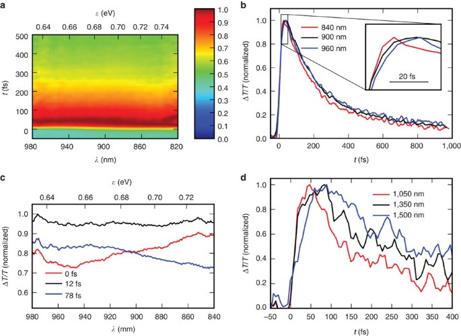Figure 2: Ultrafast transient absorption measurements. (a) ΔT/Tmap, normalized to unity, as a function of probe wavelengthλand pump-probe delayt. The scale bar ranges from 0 to 1. The positive PB signal due to Pauli blocking rises on the 10 fs timescale due to ultrafast spreading of the electron distribution upon impulsive excitation. (b) ΔT/Tdynamics at selected wavelengths of the pump-probe map. The inset shows that the onset of the signal moves to later times as the probe photon energy decreases. (c) Transient spectra at selected delays. For delays below 20 fs, the signal peaks at high photon energies due to the strongly out-of-equilibrium electron distribution. At later times (~20 fs), the signal flattens and then peaks at low photon energies, as the electron distribution thermalizes. (d) Transient dynamics at probe photon energies <1 eV. The delay in the PB onset is more evident. The recovery time slows as the electron distribution approaches the Dirac point. Figure 2a plots the two dimensional (2d) map of the differential transmission (Δ T / T ) as a function of pump-probe delay in the 1.2–1.45 eV range. Even with our time resolution, Fig. 2b shows an almost pulsewidth-limited rise of the PB signal in the near-IR. This immediately points to an ultrafast e–e relaxation, taking place over a timescale comparable to our instrumental response function. The PB signature is nearly featureless as a function of probe wavelength, as expected in SLG, given the linear energy-momentum dispersion of massless Dirac fermions (MDFs). The selected time traces at different probe energies undergo a biexponential decay, with a first time constant 150–170 fs, and a second longer one τ 2 >1 ps. As in previous studies, we assign the first decay to the cooling of the hot-electron distribution via interaction with optical phonons [16] , [17] , and the longer one to relaxation of the thermalized electron and phonon distributions by anharmonic decay of hot phonons [34] . By varying the excitation intensity we observe a linear dependence of the PB peak on pump fluence, while its dynamics is nearly fluence-independent. Figure 2: Ultrafast transient absorption measurements. ( a ) Δ T / T map, normalized to unity, as a function of probe wavelength λ and pump-probe delay t . The scale bar ranges from 0 to 1. The positive PB signal due to Pauli blocking rises on the 10 fs timescale due to ultrafast spreading of the electron distribution upon impulsive excitation. ( b ) Δ T / T dynamics at selected wavelengths of the pump-probe map. The inset shows that the onset of the signal moves to later times as the probe photon energy decreases. ( c ) Transient spectra at selected delays. For delays below 20 fs, the signal peaks at high photon energies due to the strongly out-of-equilibrium electron distribution. At later times (~20 fs), the signal flattens and then peaks at low photon energies, as the electron distribution thermalizes. ( d ) Transient dynamics at probe photon energies <1 eV. The delay in the PB onset is more evident. The recovery time slows as the electron distribution approaches the Dirac point. Full size image A deeper insight into the e–e thermalization process can be obtained from the inset of Fig. 2b , showing a delay in the onset of the PB maximum at longer probe wavelengths. In addition, by comparing Δ T / T at selected probe delays ( Fig. 2c ) we observe that, at early times (~10 fs), the spectrum has a positive slope, peaking at high photon energy. Starting from ~20 fs, it progressively flattens and changes to a negative slope, which persists and increases at longer delays. To understand the data, we recall that Δ T / T is proportional to the transient electron distribution [17] , [20] at time t . The sub-10 fs 2.25 eV pump pulse creates an electron distribution peaking at~1.12 eV above the Fermi level (red line in Fig. 5e ), while the probe-pulse samples the 0.6–0.72 eV interval. At early times, we, therefore, observe the tail of this distribution, with a positive slope. On the other hand, a thermal FD distribution, even with a typical doping usually present in as-prepared SLG (~100–200 meV) [35] , peaks at low photon energies, yielding a differential transmission with a negative slope. The transition from the non-thermal to the thermal regime, completed within~50 fs, is responsible for the change of slope of the Δ T / T spectrum. Figure 2d plots the Δ T / T dynamics measured with the second red-shifted IR probe pulse. The high temporal resolution combined with the low photon energy allows us to observe an even clearer delay in the PB peak formation. In particular, the maximum Δ T / T is reached after 40, 60 and 80 fs for probe wavelengths of 1,050 nm (1.2 eV), 1,350 nm (0.92 eV) and 1,550 nm (0.8 eV), respectively. To the best of our knowledge, this is the first experiment setting a timescale for the out-of-equilibrium carrier thermalization in SLG with a direct measurement. Tuning the probe to longer wavelengths also allows us to follow the subsequent e–ph cooling of the carrier distribution. In fact, τ 1 becomes longer (~400 fs at 1,550 nm) when probing at smaller photon energies, consistent with a distribution moving towards the Dirac point, before dissipating the excess energy into the phonon bath ( Fig. 5e ). 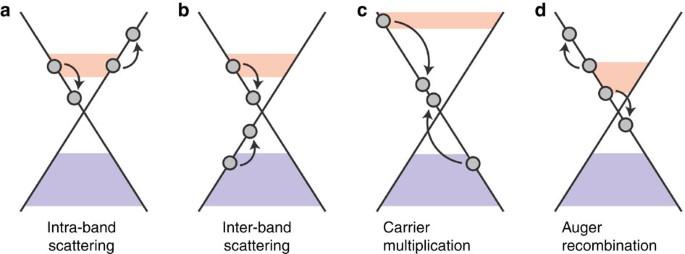Figure 3: Coulomb-enabled two-body scattering processes in graphene. Shaded areas denote occupied states, in conduction and valence band, in a non-equilibrium state, at a given time. Arrows mark transitions from initial to final states. Coulomb collisions can take place between (a) electrons in the same band (intra-band scattering) or (b) between electrons in different bands (inter-band scattering). (c,d) Electrons can also scatter from one band to the other. These ‘Auger processes’ can either (c)increase(CM) or (d)decrease(Auger recombination) the conduction-band electrons. Figure 3: Coulomb-enabled two-body scattering processes in graphene. Shaded areas denote occupied states, in conduction and valence band, in a non-equilibrium state, at a given time. Arrows mark transitions from initial to final states. Coulomb collisions can take place between ( a ) electrons in the same band (intra-band scattering) or ( b ) between electrons in different bands (inter-band scattering). ( c , d ) Electrons can also scatter from one band to the other. These ‘Auger processes’ can either ( c ) increase (CM) or ( d ) decrease (Auger recombination) the conduction-band electrons. 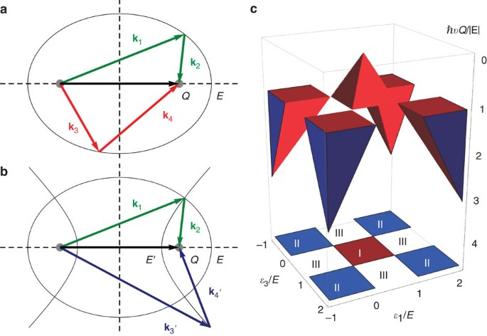Figure 4: Phase space for two-body collisions in graphene. (a) Allowed and (b) forbidden process in which two electrons with momentak1andk2scatter intok3andk4(k′3andk′4). The total momentumQ=k1+k2is conserved in both panels. Intra-band (inter-band) scattering can be represented on an ellipse (hyperbola) with distance between foci equal tov|Q|, wherevis the Fermi velocity, and the major axis equals the total energyE(E′).E=v(|k1|+|k2|) is conserved ina, which represents intra-band scattering. On the contrary, inb,E′=v(|k'3|−|k'4|) of the outgoing particles issmallerthanE. This forbidden scattering process represents a collision between two incoming particles in the same band, and two outgoing particles in different bands, i.e. an Auger process, as forFig. 3c. Energy conservation implies that Auger processes can only take place in the ‘degenerate limit’, i.e. when the vertices of the two confocal conical sections coincide with the foci. In this limit the ellipse and hyperbola collapse onto a segment and half-line, respectively, and all the momenta arecollinear. (c) The 3d solid represents the allowed values of |Q| in units ofE/(v), plotted as a function of energies ε1and ε3(both in units of total energyE) of an incoming and outgoing particle, respectively. Region I corresponds to intra-band processes; region II to inter-band processes; region III to Auger processes. No phase space is available for CM and Auger recombination for MDFs in 2d. Full size image Figure 4: Phase space for two-body collisions in graphene. ( a ) Allowed and ( b ) forbidden process in which two electrons with momenta k 1 and k 2 scatter into k 3 and k 4 ( k ′ 3 and k ′ 4 ). The total momentum Q = k 1 + k 2 is conserved in both panels. Intra-band (inter-band) scattering can be represented on an ellipse (hyperbola) with distance between foci equal to v | Q |, where v is the Fermi velocity, and the major axis equals the total energy E ( E ′). E = v (| k 1 |+| k 2 |) is conserved in a , which represents intra-band scattering. On the contrary, in b , E ′= v (| k ' 3 |−| k ' 4 |) of the outgoing particles is smaller than E . This forbidden scattering process represents a collision between two incoming particles in the same band, and two outgoing particles in different bands, i.e. an Auger process, as for Fig. 3c . Energy conservation implies that Auger processes can only take place in the ‘degenerate limit’, i.e. when the vertices of the two confocal conical sections coincide with the foci. In this limit the ellipse and hyperbola collapse onto a segment and half-line, respectively, and all the momenta are collinear . ( c ) The 3d solid represents the allowed values of | Q | in units of E /( v ), plotted as a function of energies ε 1 and ε 3 (both in units of total energy E ) of an incoming and outgoing particle, respectively. Region I corresponds to intra-band processes; region II to inter-band processes; region III to Auger processes. No phase space is available for CM and Auger recombination for MDFs in 2d. 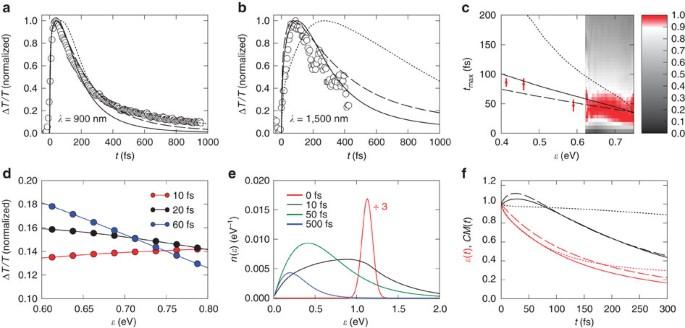Figure 5: Comparison between theory and experiments. (a) (circles) Time-evolution of ΔT/Tatnm fromFig. 2. Theoretical data from SBE using (dotted line) dynamical screening, (solid line) regularized dynamical screening and (dashed line) static screening. All data are normalized to their maximum, and correspond to a chemical potential ~200 meV (hole-doped sample). (b) As in panelafor1,500 nm. (c) Timetmax(in fs) at which ΔT/Treaches its maximum. The labelling of the theory data (lines) is the same as in (a,b). Experimental data inFig. 2aare shown as a colour plot in a continuous optical spectral range forλ≲1,000 nm. The scale bar ranges from 0 to 1. The circles with error bars correspond to three IR measurements. (d) ΔT/Tas a function of electron energy at different times. The slope inversion, signature of the initial stage of the dynamics,Fig. 2c, is correctly reproduced by theory. (e) Time-evolution of the electron population per unit cell (in units of eV−1) as derived by the SBE with regularized dynamical screening. The initial hot-electron peak (red) is centred at half the energy of the pump laser. The amplitude of this distribution is divided by 3. The hot-electron peak rapidly broadens into a non-thermal distribution (black), which then thermalises to a hot FD (green). Subsequently, cooling by phonon emission takes place (blue), until thermal equilibrium with the lattice is eventually established (not shown here since other effects neglected in our theory, such as acoustic phonons, are important in the late stages of the dynamics). When then(ε) peak energy crosses half the energy of the probe, Pauli blocking inhibits absorption. In this case a stronger transmitted PB signal is recorded at the detector. (f) CM (black curves) and CM efficiencyε(red curves), seeMethods, as functions of time. Labelling as in panels (a-c). Note the CM suppression in the prediction based on dynamical screening (black dotted line). Full size image Figure 5: Comparison between theory and experiments. ( a ) (circles) Time-evolution of Δ T / T at nm from Fig. 2 . Theoretical data from SBE using (dotted line) dynamical screening, (solid line) regularized dynamical screening and (dashed line) static screening. All data are normalized to their maximum, and correspond to a chemical potential ~200 meV (hole-doped sample). ( b ) As in panel a for 1,500 nm. ( c ) Time t max (in fs) at which Δ T / T reaches its maximum. The labelling of the theory data (lines) is the same as in ( a , b ). Experimental data in Fig. 2a are shown as a colour plot in a continuous optical spectral range for λ ≲ 1,000 nm. The scale bar ranges from 0 to 1. The circles with error bars correspond to three IR measurements. ( d ) Δ T / T as a function of electron energy at different times. The slope inversion, signature of the initial stage of the dynamics, Fig. 2c , is correctly reproduced by theory. ( e ) Time-evolution of the electron population per unit cell (in units of eV −1 ) as derived by the SBE with regularized dynamical screening. The initial hot-electron peak (red) is centred at half the energy of the pump laser. The amplitude of this distribution is divided by 3. The hot-electron peak rapidly broadens into a non-thermal distribution (black), which then thermalises to a hot FD (green). Subsequently, cooling by phonon emission takes place (blue), until thermal equilibrium with the lattice is eventually established (not shown here since other effects neglected in our theory, such as acoustic phonons, are important in the late stages of the dynamics). When the n (ε) peak energy crosses half the energy of the probe, Pauli blocking inhibits absorption. In this case a stronger transmitted PB signal is recorded at the detector. ( f ) CM (black curves) and CM efficiency ε (red curves), see Methods , as functions of time. Labelling as in panels ( a-c ). Note the CM suppression in the prediction based on dynamical screening (black dotted line). Full size image Semiclassical Boltzmann analysis The ultrashort time needed for a hot-electron distribution to thermalize is a consequence of e–e collisions [9] , [10] , [11] , [29] , [30] , [31] , [32] . We now theoretically investigate the possible Coulomb-mediated two-body collisions in SLG ( Fig. 3 ). These include intra- and inter-band scattering [10] , [11] , ‘impact ionization’ or, equivalently, ‘carrier multiplication’ (CM, i.e., increase in the number of carriers in conduction band from valence-band-assisted Coulomb scattering), and Auger recombination (i.e., decrease in the number of carriers in conduction band from valence-band-assisted Coulomb scattering). In a CM process, e.g., electrons in valence band are ‘ejected’ from the Fermi sea and promoted to unoccupied states in conduction band. CM in graphene could thus have a pivotal role in the realization of very efficient photovoltaic devices and photodetectors with ultra-high sensitivity. The findings of González et al . [9] imply that, due to severe kinematic constraints for 2d MDFs, illustrated in Fig. 4a , these processes can only take place in a collinear scattering configuration. However, it was not noticed that CM and Auger recombination processes should be nearly irrelevant in graphene as they occur in a 1d manifold (as incoming and outgoing momenta of the scattering particles lie on the same line) embedded in 2d space. Indeed, Fig. 4c demonstrates that the phase space for CM and Auger recombination in 2d MDF bands vanishes . We will return to this issue later, in connection with the calculation of the e–e contribution to the collision integral in the SBE [36] . We use this knowledge of Coulomb-mediated collisions in the framework of the SBE, the standard tool to investigate electron dynamics in metals and semiconductors [36] , [37] . We consider the equations of motion for the electron [ f s , μ ( k )] and phonon [ ] distributions, including transverse and longitudinal optical phonons at the Γ and K points of the Brillouin zone [38] , [39] , [40] . Here s =+1 ( s =−1) labels the conduction (valence) band while the valley degree-of-freedom, μ =±1, indicates whether the electron wavevector k is measured from K or K '. The electron distribution is independent of the spin degree-of-freedom. The SBE describes (i) Coulomb scattering between electrons and (ii) phonon-induced electronic transitions, where the energy of an electron decreases (increases) by the emission (absorption) of a phonon. In particular, the phonons at Γ are responsible for intra-valley transitions, while inter-valley transitions involve K phonons. Emission of optical phonons is crucial in the cooling stage of the dynamics and is possible because the photoexcited electrons energy (~1 eV) is much higher than the typical phonon one (~150–200 meV) (ref. 38 ). Finally, ph–ph interactions, arising from the anharmonicity of the lattice, are taken into account phenomenologically [30] , [32] , by employing a linear relaxation term, parametrized by a decay rate γ p h /. We neglect acoustic phonons, as they are expected to modify the electron dynamics on a timescale [34] , [41] >1 ps. Even when scattering between electrons and acoustic phonons is assisted by disorder, the so-called ‘supercollision’ process [42] , relaxation times become of the order of~1–10 ps (ref. 42 ). These are still too long compared with those considered here. We note that radiative recombination was observed either in oxygen treated graphene under continuous excitation [43] , not relevant for our case, or following ultrafast excitation in pristine graphene [44] , but with quantum efficiency ~10 −9 (ref. 44 ). We thus neglect radiative recombination. To simulate the experiments, we solve the SBE with an initial condition given by the superposition of a FD distribution in equilibrium with the lattice at T =300 K and a Gaussian peak (dip) in conduction (valence) band, centred at =±1.125 eV, with a width of 0.09 eV. The width of the pump pulse determines the width of the Gaussian peak (dip) because dephasing effects during the pump pulse, as those reported for example, in Leitenstorfer et al . [45] , contribute negligibly to the subsequent dynamics. Malić et al . [30] argued that the anisotropy introduced in the electron distribution by the pump pulse disappears in a few fs due to e–e scattering. We thus enforce circular symmetry in our SBE to deal with time-dependent distribution functions, f μ (ε k , s ), not dependent on the polar angle θ k of k , but on | k | and s =±1 only, through the MDF band energy ε k , s = sv | k |, where 10 6 m s −1 is the Fermi velocity. Thus, the e–e contribution to the SBE for the electron distribution becomes: where C μ ( ε 1 , ε 2 , ε 3 ) is the Coulomb kernel (see Methods ) describing exchange of (momentum and) energy from ε 1 and ε 2 (incoming states) to ε 3 and ε 4 = ε 1 + ε 2 − ε 3 (outgoing states) during a two-body (intra-valley) collision. Energy and momentum conservation are automatically enforced in equation (1). Circular symmetry allows us to treat the angular integrations in the Coulomb kernel analytically, taking particular care of the contributions arising from the subtle collinear scattering processes described above (see Methods ). The contribution of intra- and inter-band processes can then be cast into an integration over the allowed total momentum Q , see Fig. 4c . CM and Auger recombination require additional care. As described in Fig. 4c , their phase space in the case of 2d MDFs vanishes if momentum and energy are conserved. This statement holds true for infinitely sharp bare bands with strictly linear dispersions. Nonlinear corrections to the MDF Hamiltonian in powers of momentum (measured from the Dirac point), however, appear due to lattice effects (for example, trigonal warping) [23] . Their impact at the energy set by our pump laser is discussed in ref. 48 . Nonlinearities appear also due to the inclusion of e–e interactions [23] . These give rise to a self-energy correction to the bare MDF bands, whose real part is responsible for the Fermi velocity enhancement [25] . This correction becomes significantly large at low doping ( ≲ 10 10 cm −2 ) (refs 23 , 25 ), while here we are interested in the non-equilibrium dynamics of a substantial population of photoexcited electrons (~10 13 cm −2 ). Most importantly, any effect giving a finite width to the quasiparticle spectral function, such as e–e interactions [24] , opens up a phase space for Auger processes. To calculate the Auger contribution to C μ ( ε 1 , ε 2 , ε 3 ) we take into account these electron-lifetime effects by a suitable limiting procedure (see Methods ). We stress that the final result is independent of the precise mechanism limiting the electron lifetime. Crucially, we go beyond the Fermi golden rule by including screening in the matrix element of the Coulomb interaction at the random phase approximation (RPA) level [47] . To this end, we introduce the screened potential [47] W ( q , ω ; t )= v q / ε ( q , ω ; t ), where q and ω are the momentum and energy transfer in a scattering event, respectively, v q =2 πe 2 /( q) is the 2d Fourier transform of the Coulomb potential, is an average dielectric screening, depending on the media around the sample [23] . The RPA dynamical dielectric function is ε ( q , ω ; t )=1− v q χ (0) ( q , ω ; t ), where the non-interacting time-dependent polarization function χ (0) ( q , ω ; t ) depends on the distribution function f μ at time t : Where the prefactor 2 accounts for spin degeneracy, while the chirality factor , which depends on the polar angle θ k of k , is defined in Methods. Collinear scattering has also a key role in the theory of screening of 2d MDFs. It takes place on the ‘light cone’ ω = vq when k + q is either parallel or anti-parallel to k in equation (2). This implies a strong peak in the imaginary part of χ (0) ( q , ω ; t ) (that physically represents the spectral density of e–h pairs) close to the light cone [23] , where diverges like | ω 2 − v 2 q 2 | −1/2 . Dynamical screening at the RPA level suppresses Auger scattering. A different approximation, in which the impact of Auger processes is maximal , is the ‘static’ screening model, which consists in evaluating χ (0) ( q , ω ; t ) at ω =0. In this case, the collinear contribution to the screened potential vanishes. Note that χ (0) ( q ,0; t ) still depends on time through f μ . RPA is a very good starting point to deal with screening in metals and semiconductors [47] , but is certainly not exact. We thus modify the RPA dynamical screening function to interpolate the strength of Auger processes between its maximum (static screening) and minimum (dynamical screening). We thus introduce a third approximate screening model by cutting-off the singularity of χ (0) ( q , ω ; t ) in the region |( ω − vq )|≤Λ of width 2Λ near the light cone. This regularized polarization function, , leads to a regularized screened potential . The smearing of the singularity of the polarization function deriving from the use of the cutoff parameter Λ is a result of nonlinear corrections to the graphene band structure [46] , [48] . We stress that static and dynamical screening models are free of fitting parameters and are applicable from the IR to the optical domain. However, the theory is expected to work better in the IR limit, as it is based on the low-energy MDF Hamiltonian and thus neglects band-structure effects, which become non-negligible at high energy. We also note that Λ is a free parameter, not fixed by any fundamental constraint such as a sum-rule. In the calculations based on the regularized screening model we set Λ=20 meV without fitting the numerical results to yield the best agreement with experiments. More details on our theoretical approach and other screening models are presented elsewhere [46] . In particular, ref. 46 demonstrates that the results presented here are robust against wide changes in the parameter space. Figure 5 shows that the theory with dynamical screening compares (dotted curves in Fig. 5 ) poorly with experiments, in predicting both the prompt PB onset and its subsequent decay. While with static (and regularized dynamical) screening the calculated Δ T / T time traces are in good agreement with experiments, Fig. 5a–c , the dynamics is much slower in the presence of dynamical screening. This is best seen at low probe energies, Fig. 5b . The dependence of the Δ T / T maximum on probe wavelength, Fig. 5c , further highlights the large discrepancy between experiments and theory with dynamical screening. We trace back this discrepancy to the fact that, as stated above, dynamical screening completely suppresses Auger processes. We thus conclude that these processes are a crucially important relaxation channel for the non-equilibrium electron dynamics in graphene. Figure 5c shows that it would have not been possible to draw this conclusion without comparing theory with experiments in the low-energy regime, i.e, for energies ε <0.6 eV. Note that, even though the numerical results in Fig. 5 refer to ~200 meV p-doping, they are robust with respect to the sign of the chemical potential. This is expected, as the density of photoexcited carriers created by the pump pulse is much larger than the equilibrium carrier density. A closer inspection reveals that the thermalization of the initial hot-electron distribution, Fig. 5e , is accompanied by a very fast relaxation of the chemical potentials of conduction and valence bands, over few tens of fs. Auger processes are the only channel coupling the two bands, see Fig. 3c , and are thus responsible for this ultrafast relaxation, as e–ph scattering becomes dominant on much longer time scales of hundreds fs [14] , [15] . Thus, sufficiently hot carriers provide enough energy for the promotion of electrons from valence to conduction band, resulting in CM, as shown in Fig. 5f . CM is crucial for graphene's application in photovoltaics and photodetectors, as it can maximize the number of carriers created for a given excitation/absorption process [49] . Even though some evidence of CM was reported by Tani et al . [50] , here we experimentally access the time window and the spectral coverage where direct spectroscopic signatures of CM can be obtained. In Fig. 5f we also illustrate the ratio between the energy stored in the electronic subsystem at time t and that at time t =0 (Methods), which can be understood as the ‘efficiency’ with which the energy transferred by photons is maintained by electronic degrees-of-freedom (before being fully transferred to the lattice). As we can see from this plot, this is larger than ~50% for t <100 fs. We emphasize that dynamical screening, when cured by cutting-off the singularity of the polarization function along the light cone with the parameter Λ, improves the agreement with experiments when compared with static screening only. Indeed, the static theory underestimates screening as it misses collinear contributions to the polarization function. This explains why Δ T / T calculated with static screening: (i) increases too fast in the early stages, the electron dynamics being initially boosted by the poorly screened Coulomb repulsion, and (ii) slows down too much in the subsequent stages, when poorly screened carriers begin to accumulate close to the Dirac point. The SBE neglects intra- and inter-band quantum coherences and phase memory (non-Markovian) effects. The effect of quantum coherences can be taken into account by employing the semiconductor Bloch equations [29] or, to a greater degree of accuracy, quantum kinetic equations [37] . Including quantum coherences is expected to significantly affect the results only on the very short timescale below 10 fs (see, in particular, Fig. 5b ). Indeed, the processes that occur on the sub-10 fs timescale are not significantly affecting the overall dynamics. The striking 20 to 50 fs risetime in the PB signal at lower photon energies and the subsequent decays are sufficient to discriminate between different solutions of the SBE including or not Auger processes (see, in particular, Fig. 5c for ε <0.5 eV). These spectroscopic signatures cannot be affected by coherences. For this reason, we argue that our assessment of the importance of Auger scattering in graphene does not depend on neglecting quantum coherences in the model. A similar argument can be made about phase memory, which is also expected to persist for ultrashort time scales, comparable with the experimental resolution [51] . In conclusion, we performed time-resolved spectroscopy on SLG with an unprecedented combination of temporal resolution and spectral tunability, allowing us to track the early stages of electron thermalization. A microscopic theory based on the SBE, including collinear scattering and screening, reproduces the experiments. The ultrafast relaxation dynamics can only be explained by considering CM and Auger recombination as fundamental mechanisms driven by electron–electron interactions. We note that collinear Coulomb collisions in the intra-band scattering channel yield logarithmically enhanced quasiparticle decay rates and transport coefficients (such as viscosities and conductivities) [52] . Angle-resolved ultrafast measurements of the hot-electron distribution may shed light on these important processes. Ultrashort light pulses could be used to create a super-hot plasma of ultrarelativistic fermions (MDFs) and bosons (e.g., phonons) in graphene or in other Dirac materials, thereby creating conditions analogue to those in early universe cosmology, but within a small-scale, table-top experiment. Understanding the impact of collinear scattering on the ultrafast thermalization of MDFs can thus be of pivotal importance to achieve a deeper understanding of hot nuclear matter [53] . Graphene growth and transfer SLG is first grown on copper foils by CVD [54] . A ~25 μm thick Cu foil is loaded in a 4-inch quartz tube and heated to 1,000 °C with an H 2 gas flow of 20 cubic centimeters per minute (sccm) at 200 mTorr. The Cu foils are annealed at 1,000 °C for 30 min. The annealing process not only reduces the oxidized foil surface, but also extends the graphene grain size. The precursor gas, a mixture of H 2 and CH 4 with flow rates of 20 and 40 sccm, is injected into the CVD chamber while maintaining the reactor pressure at 600 mTorr for 30 min. The carbon atoms are then adsorbed onto the Cu surface, and nucleate SLG via grain propagation. Finally, the sample is cooled rapidly to room temperature under a hydrogen atmosphere at a pressure of 200 mTorr. The quality and number of layers of the grown samples are investigated by Raman spectroscopy [55] , [56] . The Raman spectrum of graphene grown on Cu does not show any D peak, indicating the absence of structural defects. The 2D peak is a single sharp Lorentzian, which is the signature of SLG [55] . We then transfer a 10 × 10 mm 2 region of SLG onto quartz substrates (100 μm thick) as follows [54] . Poly(methyl methacrylate) (PMMA) is spin-coated on the one side of graphene samples. The graphene film formed on the other side of Cu foil, where PMMA is not coated, is removed by using oxygen plasma at a pressure of 20 mTorr and a power of 10 W for 30 s. Cu is then dissolved in a 0.2 M aqueous solution of ammonium persulphate. The PMMA/graphene/Cu foil is then left floating until all Cu is dissolved. The remaining PMMA/graphene film is cleaned by deionized water to remove residual salt. Finally, the floating PMMA/graphene layer is picked up using the target quartz substrate and left to dry under ambient conditions. After drying, the sample is heated to 180 °C for 20 min to flatten out any wrinkles [57] . The PMMA is then dissolved in acetone, leaving the graphene adhered to the quartz substrate. A portion of the substrate is not covered with graphene, thus allowing the measurement of the nonlinear response of the substrate by a simple transverse translation of the sample. This contribution is measured to be negligible. The transferred graphene is then inspected by optical microscopy, Raman spectroscopy and absorption microscopy. After transfer, the 2D peak is still a single sharp Lorentzian, indicating that SLG has indeed been transferred. The absence of D peak proves that no structural defects are induced during the transfer process. Raman measurements over a large number of points indicate a ~200 meV p-doping [35] , [58] , [59] . Pump-probe spectroscopy The transient absorption spectroscopy set-up is driven by a regeneratively amplified mode-locked Ti:Sapphire laser (Clark Instrumentation) that delivers 150 fs pulses at 780 nm with 500 μJ energy at 1 kHz repetition rate. The laser drives three optical parametric amplifiers (OPAs), from which the visible pump pulses and the two near-IR probe pulses are generated. These are then compressed to the transform-limited duration by means of custom made chirped mirrors (visible OPA), a fused silica prism pair (IR OPA 1) and an adaptive pulse shaper based on a deformable mirror (IR OPA 2) (ref. 33 ). The pump and probe pulses are synchronized by a motorized translation stage and spatially overlapped on the sample. After the sample, the IR OPA 1 probe pulse is focused onto the entrance slit of a spectrometer equipped with a 1024 pixel linear Si photodiode array (Entwicklungsbuero Stresing). The IR OPA 2 probe pulse is instead detected by an InGaAs CCD (charge-coupled device) spectrometer (Bayspec Super Gamut). Both these devices allow a full 1 kHz readout of the spectra. By recording pump-on and pump-off probe spectra, we extract Δ T / T as a function of pump-probe delay (t) as Δ T / T ( λ , t )=[ T on ( λ , t )− T off ( λ , t )]/ T off ( λ , t ). The system has a sensitivity better than Δ T / T =10 −4 . The pump intensity is reduced to avoid any sample saturation or high-order nonlinear effects ( I pump <1 mJ cm −2 ). By moving from multichannel to single-wavelength detection, we are able to reduce the fluence by a factor 20, and observe a substantially unchanged dynamics. Δ T / T is lower than 0.007 at the PB maximum, and the signal from the substrate is found to be negligible. The density of photoexcited electrons is calculated to be 10 −13 cm −2 given the ~10 nJ pump pulse energy on a spot size of radius 80 μm, corresponding to a fluence of 50 μJ cm −2 . Semiclassical Boltzmann equation The SBE for the electron distribution, includes collision integrals due to e–e and e–ph scattering. The magnitude of the e–ph couplings is discussed in Piscanec et al . [38] , Lazzeri et al . [39] , Basko et al . [40] Here we use the values for the phonons at Γ and , for the longitudinal and transverse phonons at K , respectively. The equation for the phonon distribution, includes the collision term due to e–ph scattering and the linear relaxation with ps −1 (ref. 32 ). The equilibrium phonon distribution function consists of the Bose-Einstein thermal factor evaluated at the ν-th phonon branch , assumed dispersionless in the present treatment. This approximation is well justified as changes slowly with respect to the electron dispersion. The Coulomb kernel in equation (1) reads: where E ≡ ε 1 + ε 2 , k 2 ≡ Q − k 1 , k 4 ≡ Q − k 3 , and S is the sample area. The polar angle of k 1 does not matter, while the modulus of k 1 is equal to ε 1 /( v ). The Dirac delta distributions follow from the conservation of total energy E and momentum Q . In equation (5) we introduce the infinitesimal η in the argument of the third delta to relax energy conservation, which is restored by taking the limit η → 0. As shown in Fig. 4c , when η =0 the summand in equation (5) vanishes for Auger processes. In this case, it is important to first perform the summations over Q and k 3 , and then take the limit η →0. The squared matrix element (where the integers 1…4 indicate the dependence on s i and k i for i =1…4) includes a summation over spin degrees-of-freedom and direct and exchange [60] contributions to e–e scattering. It reads , where is the matrix element of the Coulomb interaction in the eigenstate representation of the MDF Hamiltonian [23] , with the so-called ‘chirality factor’ [23] and ω =( ε 1 − ε 3 )/. Note that Coulomb scattering occurs only within a valley μ . The contribution due to Auger processes to the Coulomb kernel can be calculated analytically: The strength of e–e interactions is parametrized [23] by the dimensionless fine-structure constant α ee ≡ e 2 /( v ). We use α ee =0.9, as appropriate for graphene with one side exposed to air and the other to SiO 2 (ref. 23 ). Δ T / T is calculated as a function of wavelength λ =2 πc / ω from the electron distribution via the following relation [20] : where is the fine-structure constant and n F ( E ) is the FD distribution. Here μ =±1 is not summed over and can be chosen at will, as the electron distribution is identical for the two valleys. The CM is calculated as: where is the electron population per unit cell in conduction band at time t , ν ( ε )=2 εA 0 /[2 π ( v ) 2 ] being the MDF density-of-states, and nm 2 the area of the elementary cell. The efficiency ε ( t ) at time t is calculated as ε ( t ) ≡ E el ( t )/ E el (0), where is the energy stored in the electronic subsystem at time t . The numerical solution of the SBE is performed with a fourth-order Runge-Kutta method. The electron energies are discretized on a mesh with a 25-meV step. The screening function and the Coulomb kernel are updated in time at multiples of the integration step, depending on the speed of the relaxation, with more frequent updates (for example, every 2 fs at the beginning of the time-evolution). The numerical results are stable with respect to changes in these choices. How to cite this article: Brida, D. et al . Ultrafast collinear scattering and carrier multiplication in graphene. Nat. Commun. 4:1987 doi: 10.1038/ncomms2987 (2013).